Rotational separation of non-spherical bioparticles using I-shaped pillar arrays in a microfluidic device Most bioparticles, such as red blood cells and bacteria, are non-spherical in shape. However, conventional microfluidic separation devices are designed for spherical particles. This poses a challenge in designing a separation device for non-spherical bioparticles, as the smallest dimension of the bioparticle has to be considered, which increases fabrication challenges and decreases the throughput. If current methods do not take into account the shape of non-spherical bioparticles, the separation will be inefficient. Here, to address this challenge, we present a novel technique for the separation of red blood cells as a non-spherical bioparticle, using a new I-shaped pillar arrays design. It takes the shape into account and induces rotational movements, allowing us to leverage on the largest dimension, which increases its separation size. This technique has been used for 100% separation of red blood cells from blood samples in a focused stream, outperforming the conventional pillar array designs. The capacity to isolate various biological entities, such as pathogen and blood components, enables the diagnosis and detection of diseases, infections and biological threats [1] , [2] . Traditional processes of separating these bioparticles, such as centrifugal separation, filtration, culture and isolation, involve cumbersome benchtop equipment. Advances in micromachining resulted in the development of microfluidic devices, in which bioparticle separation process can now be performed at microscale, commonly known as lab-on-a-chip [3] . These devices potentially have an edge over traditional techniques, as it reduces human error via automation and require low sample volumes, resulting in a rapid, high-throughput, cost-efficient and reproducible separation of bioparticles [4] , [5] . Bioparticles are separated in microfluidic devices by three general principles, namely size discrimination in sieving techniques, hydrodynamic laminar flow separation and non-inertia force fields, such as dielectrophoresis, acoustic, radiation and magnetic field [5] , [6] , [7] , [8] . The main separation criteria for all these methods depend on the spherical diameter of these bioparticles (that is, particles are considered as spherical) [5] , [9] . Dependence on the spherical size poses a challenge for the separation of non-spherical bioparticles. Biological entities, such as rod-shaped bacteria and disc-shaped red blood cells (RBCs), have disproportional length and width, which complicates the separation process designed for spherical particles, as the narrowest width has to be considered for the separation criteria within the design parameters of the microfluidic devices. One of the clinically relevant non-spherical bioparticles is the RBC, as its separation from plasma allows diagnosis of different diseases. RBCs are disc-shaped biconcaved cells with a diameter of ~8 μm and thickness of about 2 μm. Separation techniques, such as RBC flow margination, cross-flow filtration and deterministic lateral displacement (DLD) have been used for RBC separation from whole blood [1] . RBC flow margination technique utilizes the difference in size and deformability of RBC and other circulating cells for the separation. The deformable RBCs migrate to the center of the fluidic channels, while the larger white blood cells or smaller bioparticles, such as platelets or bacteria, migrate to the walls of the channel. Multiple RBC cell margination flow iterations have enabled purification of RBCs from bacteria and leukocytes, while malaria-affected cells were separated with an efficiency of ~75–90%, depending on its stage of infection [10] , [11] . Hou et al . [10] , [11] also briefly mentioned that the non-spherical shape of bacteria could have contributed to the separation process, which emphasizes the impact of shape-based sorting. Cross-flow filtration techniques were also used to separate RBC and plasma where the blood sample flows within a straight channel, while the plasma or smaller particles elute out of the sample using narrow pores or channel gaps aligned perpendicular to the flow [9] . VanDelinder et al . [12] and Crowley et al . [13] both designed a cross-flow gap size of 0.5 μm to prevent RBCs from migrating past the gaps. DLD devices have also been used to separate RBCs from blood and plasma, which allows distinct separation into separate streams [14] , [15] , [16] . To effectively separate the RBCs, it is assumed to have a critical separation diameter of 2 μm to compensate for deformation or possible preferential orientation of RBCs at its thinnest dimension in the laminar flow stream. Recent developments for RBCs separation in DLD devices control the orientation of RBCs by reducing the channel depth to a minimum, allowing an increased separation diameter [14] , [17] ; however, this confines the sample to a narrow channel depth, which restricts high throughput and is not necessarily effective for other non-spherical particles, such as rod-shaped or spiral-shaped bacteria. These separation techniques do not provide a comprehensive solution for the separation of non-spherical particles. Hence, to effectively separate non-spherical biological entities for rapid medical diagnosis, new separation methods, which take into consideration the multivariate shapes of the bioparticles, are required. Here we present a novel separation technique taking into account the shape of the particles by inducing continuous rotation of the particles. This separation principle is based on DLD, which has been established as an efficient technique for the continuous-flow separation of particles that are dependent on their spherical dimension, by using conventional cylindrical pillars [18] , [19] , [20] , [21] . Accounting for the shape of particles, we hypothesize that inducing rotations of non-spherical particles will increase the effective separation size of the particles. By leveraging on the continuous rotation of a non-spherical particle, we are able to reduce the emphasis on the narrowest width and instead focus on mimicking a spherical particle based on its greatest length. From our hypothesis, we have designed a novel I-shaped pillar to induce the rotation of non-spherical particles flowing in the laminar stream through our separation device shown in Fig. 1a . The pillar shape and principle is schematically explained in Fig. 1b with the example of a disc-shaped particle. The critical diameter of the particle to be separated in Fig. 1b (i) would be the smallest dimension of the particle ( D 1 ) while the rotating disc-shaped particle in Fig. 1b (ii) would have a maximum rotational diameter of D 2 , which is much greater than D 1 . The I-shaped pillar has two protrusions, which induce rotations, and a middle groove to accommodate the rotation. By inducing continuous rotation and by increasing the effective size for separation, our novel design can potentially separate the bioparticles with diverse shapes and sizes. 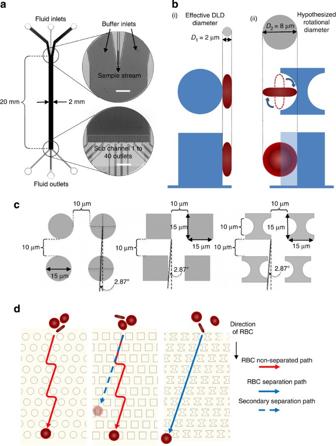Figure 1: Schematics of device designs and hypothesis. (a) The sample stream is sandwiched between two buffer streams, and the output channels are divided into 40 subchannels for quantification of the RBC separation process. White scale bar, 250 μm. The hypothesis schematics inbshows the difference between the conventional DLD pillars in (b, i) and I-shaped DLD pillars in (b, ii) with both top view and cross-section view at the bottom. Three devices of fixed DLD parameters and varying shape is shown inc, namely cylindrical, square and I-shaped pillar array. Lastly,dit depicts the projected paths of RBCs, as it flows within the respective devices. Figure 1: Schematics of device designs and hypothesis. ( a ) The sample stream is sandwiched between two buffer streams, and the output channels are divided into 40 subchannels for quantification of the RBC separation process. White scale bar, 250 μm. The hypothesis schematics in b shows the difference between the conventional DLD pillars in ( b , i) and I-shaped DLD pillars in ( b , ii) with both top view and cross-section view at the bottom. Three devices of fixed DLD parameters and varying shape is shown in c , namely cylindrical, square and I-shaped pillar array. Lastly, d it depicts the projected paths of RBCs, as it flows within the respective devices. Full size image Some efforts have been made to change the post shape of DLD to enhance its critical separation diameter [22] , [23] . Loutherback et al . [22] , [23] have demonstrated that by using triangular pillars, the flow profile becomes asymmetric, resulting in a reduced critical diameter as compared with conventional DLD. However, this improvement does not address the varying critical diameter of a non-spherical particle. Sugaya et al . [24] have also observed that by rotating non-spherical particles at the T-junction in a hydrodynamic filtration device, separation of non-spherical particles based on its longer dimension can be achieved. However, it is limited to a single flipping event of a non-spherical particle at the T-junction, which determines the success or failure of the separation process. Here we study the effect of novel I-shaped pillar on the continuous rotation and, hence, the separation of disc-shaped RBCs. The novelty of our project is twofold. First, we successfully separated non-spherical particles by inducing continuous rotations. Second, we present a novel design in terms of I-shaped pillar for the induction of rotations and, hence, separations of these particles in a laminar flow separation process. Our current findings for RBCs separation could potentially separate other non-spherical particles, like pathogens, with higher-throughput and efficiency, circumventing the spherical size dependency of current techniques. RBC separation and comparison study The novel I-shaped pillar design can induce rotations for non-spherical particles to increase the RBC’s effective separation size. The term ‘effective separation size’ is referred here as the critical diameter of particle needed for separation in our device. Figure 1d shows comparison of RBC separation paths between cylindrical pillars, square pillars and I-shaped pillars. All three pillar types in Fig. 1c are designed with exactly the same DLD dimensions of 10 μm gap size, pillar shift gradient of 2.86 o and a maximum pillar length of 15 μm. The device was etched to ~15 μm deep. We wanted to compare how the conventional cylindrical pillars fared with sharp edges of square pillars and the proposed I-shaped pillars. The overall device setup can be seen in Supplementary Fig. S1 . There are 40 output subchannels identified as channel 1–40 starting from left to right shown in Fig. 1a . To quantify the effect of separation, RBCs at each subchannel output is counted and is tabulated as a ratio of the total RBCs calculated. However, only channels 1–30 is tabulated in the graph shown in Fig. 2 , as there are no RBCs flowing in channels 31–40 due to the buffer stream on the right side of the graph. In all three pillar types, fresh blood is infused into the device using a syringe pump at a rate of 0.2 μl min −1 . The buffer streams sandwich the sample stream with a flow rate of 0.5 μl min −1 each. At these flow rates, the input distribution of RBC for the sample stream spreads from channel 17 to channel 26 (see Supplementary Fig. S2 ). The result for output stream is shown in Fig. 2 , which concurs with the schematics shown in Fig. 1d . Clearly shown are the RBC separation at the output regions with minimal RBC separation for cylindrical pillars in Fig. 2a , scattered distribution of RBC for square pillars in Fig. 2b and highly effective and focused separation for I-shaped pillars in Fig. 2c . Three sets of video output data were acquired using the high-speed camera, and the ratio of RBCs at the output were tabulated into the graphs ( Fig. 2 ). 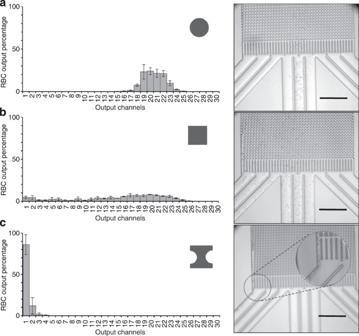Figure 2: RBC separation at output channels. Results of the RBC separation for cylindrical pillars (a), square pillars (b) and I-shaped pillars (c). The histograms are plotted by the percentage of total RBC at the output channels. The screen capture of the output regions are shown on the right of the respective graphs. (c) Magnified region of the I-shaped DLD pillars at the output channels 1–5. All error bars were calculated as s.d. at individual outputs of three samples taken from three experiments. Scale bar, 250 μm. Figure 2: RBC separation at output channels. Results of the RBC separation for cylindrical pillars ( a ), square pillars ( b ) and I-shaped pillars ( c ). The histograms are plotted by the percentage of total RBC at the output channels. The screen capture of the output regions are shown on the right of the respective graphs. ( c ) Magnified region of the I-shaped DLD pillars at the output channels 1–5. All error bars were calculated as s.d. at individual outputs of three samples taken from three experiments. Scale bar, 250 μm. Full size image RBC separation is not observed in the cylindrical pillar array for the given parameters. The final output shown in Fig. 2a depicts the RBC output distribution ratio to be between channels 15 and 25, which do not deviate from the original sample distribution of channels 17–26. The distribution peaked at ~24% in channel 20. The critical diameter of the cylindrical pillars is calculated to be 3.33 μm, based on the recent DLD blood separation papers, which simplify the original formulation for critical diameter calculations (see Methods) [14] , [16] , [17] , [19] . For DLD separation to be effective, the particle to be separated has to be larger than the critical diameter. In this case, the RBC’s narrowest width (2 μm) is smaller than the critical diameter, resulting in no separation that can be seen in the distribution of RBC ratio in Fig. 2a . From Fig. 2b , the RBC separation in square pillar array shows a widely distributed RBC output ratio ranging from channels 1 to 26. The peak RBC output ratio is ~8% at channel 20. Though 63% of the RBC is distributed near the central regions (between channels 15 to 25), there are RBCs that deviated all the way to channel 1. Comparatively, square pillar have an effect on RBC separation as compared with cylindrical pillars with the same pillar array parameters, such as gap size (10 μm) and pillar array gradient (2.86 o ). It is important to note that the RBCs do rotate in the square pillar array. From Fig. 3a , we can see that the edge could have caused the RBC to flip and rotate. This could have an effect on the separation, causing a widespread of RBC distribution ratio shown in Fig. 2b . Although this result in square pillars requires further investigation, our main focus is to use it as a control for I-shaped pillars. The distinct spread and scattering of RBC distribution for square pillars show that the square pillar array has an enhanced effect on RBC separation compared with cylindrical pillars, but not effective enough to ensure an efficient separation. In contrast to square and cylindrical pillars, I-shaped pillars are extremely effective in separating RBCs. The output graph in Fig. 2c shows complete separation of RBC in channels 1–4, deviating away from its original RBC input distribution of channels 15–26. Also, the peak distribution of ~86% in channel 1 is distinctly greater than the peak distribution for square (~8%) and cylindrical pillar (~24%) array devices. The slight spread to channels 2 and 3 are due to slight overcrowding of RBC in channel 1, which spill over to the other channels. The magnified view shows a snap shot of the 100% separated RBC stream in the output channel 1 ( Supplementary Movie 1 ). This focused stream of RBC separation clearly shows the effectiveness of I-shaped pillars compared with the control square pillar array and the conventional cylindrical pillar array. As the pillar array gap size and gradient are fixed across the three pillar types, it would suggest that the effective separation size of RBC in I-shaped pillar array is greater than square pillars and cylindrical pillars. 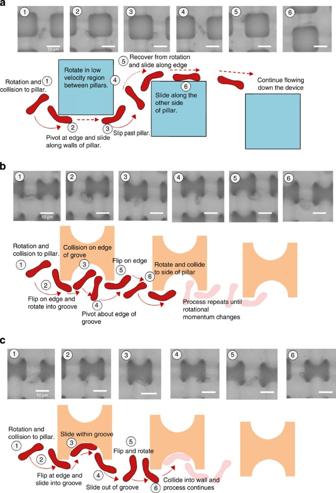Figure 3: RBC movement within square and I-shaped pillars. The major RBC flow movement within the square pillar array (a) and the I-shaped pillars (b,c) are depicted in the form of schematics, as well as video still capture. (a) Primary movement of RBCs in square-shaped pillars in six steps shown in the video still capture as it flows down the non-separated path. (b,c) RBC separation path with two types of observed rotational movements within the I-shaped pillars. Scale bar, 10 μm. Figure 3: RBC movement within square and I-shaped pillars. The major RBC flow movement within the square pillar array ( a ) and the I-shaped pillars ( b , c ) are depicted in the form of schematics, as well as video still capture. ( a ) Primary movement of RBCs in square-shaped pillars in six steps shown in the video still capture as it flows down the non-separated path. ( b , c ) RBC separation path with two types of observed rotational movements within the I-shaped pillars. Scale bar, 10 μm. Full size image Bead characterization of the I-shaped device To confirm our hypothesis that I-shaped pillar is more effective for non-spherical RBC, we characterized the critical separation diameter of the I-shaped pillar device and investigated the critical size of a rotating RBC in the I-shaped pillar array. The separation results of the beads in I-shaped pillar and cylindrical pillar devices are shown in Supplementary Fig. S3 . National Institute of Standards and Technology polystyrene beads of size 2.0–3.5 μm in steps of 0.5 μm were used as the lower and upper limits of the test. Two micrometre and 2.5 μm beads were not separated in the conventional DLD device (see Supplementary Fig. S3a). However, slight separation was observed for 3 μm beads, for which the output separation channels ranged from channel 8 to 22 with a peak separation of ~26% at channel 18. Though the spread of 3 μm is wide, 85% of the separated beads lie close to the centre regions of channel 14–22. The actual critical diameter of the conventional DLD pillar array is between 3 and 3.5 μm, which concurs with the theoretical critical diameter of the device 3.33 μm. I-shaped pillars on the other hand do not have a well-established study of its theoretical critical diameter. From the bead flow tests, it is interesting to note that although 2 μm beads were not separated, there was distinct separation for 3 μm beads and significant deviation of 2.5 μm beads at the output regions (see Supplementary Fig. S3b and Supplementary Note S1 ). Beads (2.5 μm) peaked at ~16±1.7% separation at channel 6, whereas the output distribution spread was wide and relatively evenly distributed along channels 4–15. The spread that is observed here seems counter-intuitive to the previous performance of DLD devices, which enables distinct separations [18] , [21] , [25] . The observed phenomenon could be due to DLD mixed separation mode and further elaborated in Supplementary Note S1 ( [26] , [27] , [28] ). From the results, the effective critical diameter of the I-shaped device can be experimentally deduced to be greater than 2.5 μm and less than 3 μm for distinctive particle separation. RBC rotational movement To investigate the influence of RBC rotation on the increase in effective separation, the movement of RBCs in both square pillar in Fig. 3a and I-shaped pillar array in Fig. 3b are captured and analyzed (see Supplementary Movies S2 and S3 ). Detailed schematics and screen shots of the motion of RBC within the square control and I-shaped pillar are described in Fig. 3 . Figure 3a depicts the path of RBC, which does not get separated in square pillars. The RBC’s movements follow a laminar flow path and flow length-wise close to the side of the pillars; hence, the effective separation diameter of the RBC is ~2 μm, which is the width of the RBC. It is also noted that as it collides into the walls of the pillar in step 1 in Fig. 3a , it deforms and conforms to the shape of the pillar, sliding along the walls. During the collision and deformation process in steps 1 and 2 in Fig. 3a , if the RBC does not slide close to the walls of the pillar, it might get displaced from its original laminar flow path (bumped) and get separated. RBC itself is a compliant and deformable object; hence, it is hard to predict its movement in a post-collision scenario within a complex fluid flow. Although majority of the RBCs in the square pillar array slides along the pillar unaffected, some of them would be displaced due to the randomness of their rotation. This would result in a possible bumping and, hence, some separation as observed in the square pillar array, explaining the spread of RBCs throughout the output channels. Figure 3b and c shows two observed motions of RBCs, as they flow past I-shaped pillars. These two figures depict the motion of a RBC that allows it to follow the gradient of pillar array resulting in the final displacement from the original laminar flow path and hence separation at the output channels. Figure 3b shows a bumping and tumbling motion, whereas Figure 3c shows RBC sliding motion along the sides of the wall, which is similar to the schematics shown for the RBC movement in square pillar array. However, the key difference that enables RBC separation lies in the I-shaped protrusions, which prevent the RBC from taking the usual streamline path by flipping it as it exits the groove of the pillar. Though both types of RBC movements in Fig. 3b and Fig. 3c differ, the I-shaped protrusions act as a two pivot points for the RBC to rotate, and the groove provides room for RBC to flip and tumble within (steps 1 and 4 in Fig. 3b and c ). Both RBC movements are not mutually exclusive and can alternate between Fig. 3b and c separation processes. This distinct difference in RBC movement compared with the square pillar shows how a simple groove in the novel I-shaped pillar design would destabilize the streamline flow of the RBC and allow it to flip and rotate, resulting in increased effective size for separation. Hence, the I-shaped pillar have shown to induce rotations of RBC, resulting in a greater effective separating size proposed in our hypothesis. Computational fluid dynamic To have a basic understanding on how the I-shaped pillars would have induced rotations of RBC, we performed computational analysis on COMSOL Multiphysics 4.1 platform for the square pillar array and I-shaped pillar array to study the fluid flow and velocity profile. We wanted to find out what fluid flow conditions would the RBC experience in our devices. For the computation of each device, we have set a simple setup of a minimum two by two pillar array and the initial flow velocity is set to 1 mm s −1 with atmospheric pressures at the outlets. All boundary conditions were set the same for both models. The computational data in Fig. 4 shows the velocity and streamline profile for both devices. It can be seen that square pillars in Fig. 4a have relatively constant and smooth fluid streamlines between the pillars, unlike I-shaped pillars in Fig. 4b where the groove between pillars causes a disturbance in peak velocity streamline path. The superimposed RBCs in both figures are placed in the similar positions that can be seen in Fig. 3a (step 2 and 3) and Fig. 3b (step 4 and 5). The RBC in Fig. 4a is placed to mimic a sliding RBC. The graph in Fig. 4c shows the fluid velocity flow across the length of the superimposed RBC, as it slides along the walls of the square pillar. The flow velocity does not fluctuate when the RBC is in that position. This would support the observation of a sliding RBC. 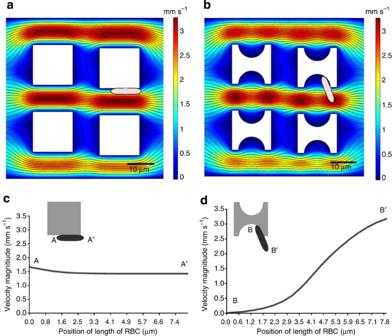Figure 4: COMSOL multiphysics fluid flow simulation for square and I-shaped pillars. Comparison of fluid flow profiles of square pillars (a) and I-shaped pillars (b) can be seen in the simulated flow patterns. Red regions represent high flow rates of ~3.5 mm s−1while dark blue represents zero flow at the no-slip boundary condition. The superimposed elongated rod-shaped figure in light pink is used to represent the position of RBC in the fluid flow experiencing different velocities across the RBC body. The graph incanddshows the cross-section fluid flow magnitude experienced by the RBC at its superimposed position inaandb, respectively. Figure 4d depicts an RBC, which is transiting from step 4 to step 5 as shown in Fig. 3b . In contrast, it shows a drastic variation in flow velocity across the RBC, which has a high (3.2 mm s −1 ) to a low (close to 0) flow rate. The RBC in such a position depicted in Fig. 4b would experience a deferential flow velocity, resulting in the formation of a net moment acting on the RBC, causing it to rotate. The double protrusions in I-shaped pillar compliment the groove by creating variations in fluid streamlines and velocities producing changes in moments on the RBC, hence the observed RBC’s rotation and separation in our novel design. Although the I-shaped pillar proves more effective for non-spherical RBCs, it maintains a symmetrical cross-sectional fluid flow profile and differs from other unique DLD pillar shape, such as triangular shape, with asymmetrical fluid flow profile (see Supplementary Fig. S4 and Supplementary Note S2 ) [23] . Figure 4: COMSOL multiphysics fluid flow simulation for square and I-shaped pillars. Comparison of fluid flow profiles of square pillars ( a ) and I-shaped pillars ( b ) can be seen in the simulated flow patterns. Red regions represent high flow rates of ~3.5 mm s −1 while dark blue represents zero flow at the no-slip boundary condition. The superimposed elongated rod-shaped figure in light pink is used to represent the position of RBC in the fluid flow experiencing different velocities across the RBC body. The graph in c and d shows the cross-section fluid flow magnitude experienced by the RBC at its superimposed position in a and b , respectively. Full size image I-shaped pillars have shown to have an increase in separation effectiveness for non-spherical RBCs and it has also reduced the device critical diameter for I-shaped pillars to less than 3 μm. Further testing was performed to test whether the separation of RBC in I-shaped pillars was due to the reduction of device critical diameter or increase in rotational diameter as hypothesized in Fig. 1b (see Supplementary Fig. S5 and Supplementary Note S3 ). The RBC rotational diameter was characterized and found to have increased to ~3.5 μm and, hence, would confirm that the observed separation in I-shaped pillars was due to an increase in RBC critical diameter. Further testing on increasing flow velocity of up to ten times has shown that the I-shaped pillar remained effective in the separation of non-spherical RBCs with separation critical diameter of more than 3 μm (see Supplementary Fig. S6 and Supplementary Note S4 ). To further extend our hypothesis, we briefly tested the effects of I-shaped pillars on other non-spherical particle, such as the rod-shaped bacteria, and have found that it was also effective in the separation of the Escherichia coli bacteria. The preliminary studies on extended applications of I-shaped pillar array for rod-shaped bacteria separation resulted in the displacement of a bacteria stream path with a critical diameter of 1.12 μm, which is approximately half of the length of the E. coli bacteria (see Supplementary Fig. S7 and Supplementary Note S5 ). Conventional DLD pillar arrays were not able to separate the bacteria at those parameters. Currently, separation of bacteria using DLD has not been performed and there are no current comparisons for the DLD study. We have introduced a novel I-shaped pillar array for the separation of non-spherical bioparticles, such as RBC and E. coli . Our results and computational studies have shown that the I-shaped pillar destabilizes the laminar flow movement of RBC and induces rotation, which supports our hypothesis to enable the effective separation of the disc-shaped RBCs from the sample stream as compared with the conventional cylindrical pillar and square pillar array. Our studies with I-shaped pillar differ from past works in two aspects (see Supplementary Discussions ). First, the pillar design and mechanisms for particle separation differ greatly, as we aim to induce continuous rotation and have shown that the rotation and tumbling of disc-shaped RBCs by I-shaped pillar array would result in a focused separation stream. Second, we enable an increase in particle critical diameter by accounting for the shape of particle to be separated from leveraging on its maximum length in a continuous rotation. To conclude, the I-shaped pillar array has been proven to be more effective in the separation of non-spherical bioparticles compared to current particle separation techniques by using the RBCs and E. coli bacteria as proof-of-concepts for the potential separation of the vast number of non-spherical biological entities, such as bacteria, fungi and, maybe, even viruses. Device fabrication The device design shown in Fig. 1a comprises three inlet channels, a pillar-array main channel of 2 cm long and three outlet channels divided into 40 subchannels for characterization of device separation efficiency. There are a total of three pillar array designs as shown in Fig. 1c , namely cylindrical pillar, square pillar and the I-shaped pillar. All calculations of DLD were based on formula used by Davis et al . [16] , as all recent works on RBC separation in DLD devices were designed from the proposed model. As such, all devices used in the paper were based on: where D C =critical diameter, g =gap size between pillars and N =number of rows per shift in columns (that is tan −1 (1/ N )=gradient of pillar array). The designs of the device were drawn on AutoCAD and sent for a chrome-glass mask (Infinite Graphics, Singapore) fabrication. Fabrication of the device was performed in Institute of Materials Research and Engineering in a clean room. The silicon microfluidic device was fabricated on a silicon wafer using standard photolithographic and dry etching techniques. The device design in Fig. 1a was transferred from a glass mask to a positive photoresist (AZ5214E, Microchem, MA) coated on the silicon surface by photolithography followed by deep reactive ion etching to a depth of 15 μm. A thin sheet of poly-dimethylsiloxane (PDMS, Dow Chemicals, MI) was fabricated, and the inlet and outlet holes were punched before this PDMS sheet was bonded over the silicon device, using oxygen plasma (see Supplementary Fig. S1a ). AZ5214E (Microchem, MA)-positive photoresist was spin coated on the silicon wafer at 4,000 r.p.m. (rounds per minute) for 1 min and baked at 95 °C for another min. The patterns were transferred to the photoresist using a SUSS MA8 photolithography machine. The patterns were developed and hard baked at 125 °C for a minute. Oxford 180 dry reactive ion etching machine was used for the fabrication of the pillars. A total of 25 cycles of Bosch etch techniques were performed, with each etch of ~0.6 μm per cycle. After the dry etching, the remaining photoresist was removed with acetone, washed for 1 min and dipped in AZ300T (Hoechst, NJ) photoresist stripper for 10 min at 80 °C. It is finally rinsed with deionized water. The PDMS (Dow Corning, MI) cover shown in Fig. 1a was initially mixed with a ratio of 10:1 of polymer and curing agent. The mixture was poured into a flat glass mould and was degassed for 30 min and baked at 75 °C for 45 min. Rectangular pieces of ~2 cm by 4 cm were cut and holes of 0.5 mm diameter holes were punched on the PDMS cover. An oxygen plasma machine was used to activate the surface of both the silicon and processed PDMS before aligning the holes to the channels of the device. The final device was placed overnight to allow the PDMS to bond to silicon properly. RBC separation The inlet tubes were attached to the final device and washed with 1% w/v pluronic F127 (Sigma Aldrich, Singapore) in deionized water for 30 min. This is for surface passivation to prevent any form of non-specific attachment of the sample. The blood sample was extracted from a finger prick and diluted ten times in 1 × PBS buffer (Sigma Aldrich, Singapore). The diluted blood sample was driven by using a syringe pump at a flow rate of 0.2 μl min −1 and sample PBS buffer streams at a flow rate of 0.5 μl min −1 . The high-speed video footages on the motion of RBCs were captured by Phantom Miro M310 at frame rates ranging from 250 to 3,000 frames per second. These raw videos were analysed, and results were tabulated and shown in Figs 2 and 3 . The output data was compiled by counting and averaging the total number of cells at various output channels for three devices per experiment set. All videos were uncompressed into a real-time video of 60 s. The motion of the particle was slowed by 40 times to allow counting of the number of particles at the outlets. Three videos were captured to get an average number of particle distributions over the subchannels. Though there are no specific subchannels for input, the total number of output channels coincided with the total number of pillars in a horizontal width of the channel, which allowed the tabulation of RBC input distribution. Screen shots were extracted to view the motion and position of RBCs for its interaction with the pillars. Video footages can be found in the Supplementary Movies provided with this manuscript. How to cite this article: Zeming, K. K. et al . Rotational separation of non-spherical bioparticles using I-shaped pillar arrays in a microfluidic device. Nat. Commun. 4:1625 doi: 10.1038/ncomms2653 (2013).